Cortical responses elicited by photovoltaic subretinal prostheses exhibit similarities to visually evoked potentials We have previously developed a wireless photovoltaic retinal prosthesis, in which camera-captured images are projected onto the retina using pulsed near-IR light. Each pixel in the subretinal implant directly converts pulsed light into local electric current to stimulate the nearby inner retinal neurons. Here we report that implants having pixel sizes of 280, 140 and 70 μm implanted in the subretinal space in rats with normal and degenerate retina elicit robust cortical responses upon stimulation with pulsed near-IR light. Implant-induced eVEP has shorter latency than visible light-induced VEP, its amplitude increases with peak irradiance and pulse duration, and decreases with frequency in the range of 2–20 Hz, similar to the visible light response. Modular design of the arrays allows scalability to a large number of pixels, and combined with the ease of implantation, offers a promising approach to restoration of sight in patients blinded by retinal degenerative diseases. Retinitis pigmentosa (RP) is the leading cause of inherited blindness in the young population, and currently there is no effective treatment. Age-related macular degeneration (AMD) is the major cause of vision loss in people over 65 years in the Western world [1] . Development of wet-type AMD and associated vision loss can be slowed down using monthly injections of anti-VEGF agents [2] , [3] , but there remains no cure, as there is no treatment for the dry form of AMD. As the life expectancy increases, the age-related vision loss is becoming a critical issue. National Eye Institute estimates nearly 3 million people in the United States will have moderate to severe vision loss due to retinal degenerative diseases by 2020 (ref. 1 ). In these blinding conditions, photoreceptors degenerate, yet the inner retinal neurons (inner nuclear and ganglion cell layers) that process the visual signals and relay them to the brain are relatively well preserved [4] , [5] , [6] . Patterned electrical stimulation of the inner retinal neurons can elicit pattern perception, thereby restoring sight to some degree, as was recently demonstrated in clinical studies [7] , [8] . There are several strategies to transfer visual information to the blinded retina, the two major ones are electrical stimulation of retinal neurons with electrode arrays positioned either epiretinally or subretinally. Excitation of retinal ganglion cells (RGCs) by electrodes positioned on the epiretinal surface bypasses inner retinal circuitry and requires high-frequency stimulation to elicit burst responses [9] , [10] . Recently, an epiretinal implant with 5 × 5 mm array of 60 electrodes has been approved for clinical use in Europe (Argus II, Second Sight Inc., CA). The group reported successful implantation in 30 patients with a best visual acuity of 20/1260 (ref. 7 ). As epiretinal electrodes are positioned on top on the nerve fibre layer and axonal stimulation thresholds are similar to that of RGC somas [11] , axonal stimulation is hard to avoid. It is likely the cause of arcuate or wedged visual percepts in patients stimulated with single epiretinal electrodes [12] . Current studies are aiming at development of selective targeting of ganglion cells using more sophisticated stimulation protocols [13] . Implantation of the system including the extraocular receiving coil and signal-decoding electronics box connected to the retinal stimulation array via trans-scleral cable is rather complex, with 30% of patients reporting implant-related complications [7] . Scaling such an approach to a much larger number of pixels is challenging. Although surgically more invasive, placement of electrodes into the subretinal space to stimulate bipolar cells has the potential advantage that the electrical pulse is processed by retinal circuits, converting it into the more natural bursting patterns of the RGCs. This approach is adopted by several groups, including Retina Implant AG, where a subretinal video camera having 1,500 pixels (70 μm in size) is used to convert images into local electric current in each pixel, to stimulate the retina [8] . Power is provided via a cable that exits the eye, and is routed under the skin to behind the ear. A transdermal magnetic coupler delivers the power to the receiver, as in a cochlear implant [14] , [15] . In the first clinical trial, the company reported visual acuity of up to 20/1200 (ref. 8 ), and more recently up to 20/550 (ref. 16 ), still significantly lower than would be expected from the pixel density. This could be attributed, at least in part, to the pixel cross-talk resulting from the monopolar electrode design sharing common remote return electrode [17] , [18] . In addition to high pixel density, a major advantage of this system is in the photosensitive nature of the implant, obviating the need for an external video camera to capture the images. Disadvantages of the device include a complex surgery involving many structures of the eye, the orbit and the skull and a limited dynamic range of ambient illumination enabling normal operation of the intraocular camera. Peripheral vision is often preserved in AMD patients, which helps maintain their visual acuity at the level of about 20/400, with off-centre fixation. This major group of low-vision patients would benefit from a retinal prosthesis if it would provide visual acuity of about 20/200 or better. Our approach is photovoltaic and subretinal [19] . Images of the visual scene acquired by video camera are processed and projected by video goggles onto a subretinally placed photodiode array using pulsed near-IR (~900 nm) light. Photovoltaic pixels in the array convert pulsed light into biphasic pulses of electric current that stimulate retinal neurons (primarily in the inner nuclear layer, INL). This system offers several advantageous features: thousands of pixels in the implant can be activated simultaneously and independently; as the pixels are activated by light, no wires are involved, which greatly simplifies the surgical procedure; an external camera allows operation over a wide range of ambient illumination and provides user-adjustable image processing; the optical nature of the device maintains the natural link between eye movements and image perception; modular implant design allows implantation via a small retinotomy, while tiling permits expansion of the stimulated field. Several prototypes of the photodiode array were developed based on prior experimental and theoretical work [20] , [21] , [22] with pixel sizes of 280, 140 and 70 μm and corresponding electrode diameters of 80, 40 and 20 μm ( Fig. 1 ). Each pixel is composed of three photodiodes in series, connected between the active and return electrodes [19] , [23] . As the photovoltage of each silicon diode is limited to about 0.5 V, three photodiodes in series produce stimulation voltage within the safe ‘water window’ (electrode polarization between −0.6 and +0.8 V on active and return electrodes), thus avoiding water electrolysis and electrode erosion [20] , [21] . In vitro studies of retinal stimulation with these arrays demonstrated stimulation thresholds ranging from 0.3 to 0.9 mW mm −2 with pulses from 4 to 1 ms in duration, respectively [19] . Encouraged by these results, we assessed the in vivo retinal response to chronically implanted photodiode arrays in rats with normal and degenerate retinas. 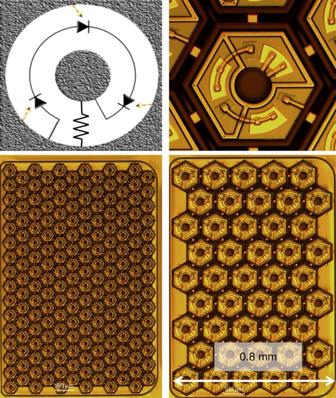Figure 1: Photovoltaic implants. Upper left: diagram of a single pixel, including three photodiodes in series connected between the active central and peripheral return electrodes. Upper right: light microscopy of a 140-μm pixel in the array. Lower panels: 0.8 × 1.2 mm photodiode arrays with 70 μm pixels (left) and 140 μm pixels (right). Figure 1: Photovoltaic implants. Upper left: diagram of a single pixel, including three photodiodes in series connected between the active central and peripheral return electrodes. Upper right: light microscopy of a 140-μm pixel in the array. Lower panels: 0.8 × 1.2 mm photodiode arrays with 70 μm pixels (left) and 140 μm pixels (right). Full size image We found that photovoltaic implants are well tolerated in subretinal space, and elicit robust cortical responses, with shorter latency than the visible light-induced responses. Amplitude of the cortical response increased with peak irradiance and pulse duration, and decreased with frequency in the range of 2–20 Hz, similar to the visible light response. Ease of implantation, scalability to a large number of pixels and simplicity of optical activation of the subretinal photodiode arrays enhance the appeal of photovoltaic approach to restoration of sight in patients blinded by retinal degenerative diseases. Array resolution For rat eye implantations, we produced arrays of 0.8 × 1.2 mm in size, containing 13, 45 and 186 pixels of 280 μm, 140 μm and 70 μm in width, respectively ( Fig. 1 ). A local return electrode in each pixel helps confine electric current in front of each pixel, an essential feature for high-resolution stimulation. High-charge injection is achieved using iridium oxide coating of the electrodes [21] . Light reflection from the device is minimized using an antireflection coating consisting of 60 nm of SiO 2 and 70 nm of SiN x . The pixel density with 70 μm pixels is 209 pixels per mm 2 , corresponding to more than 4,800 pixels over an area similar to the ARGUS II implant of Second Sight Inc. (5 × 5 mm). Anatomy of subretinal implantation Eight arrays with pixel sizes of 280 μm, 9 with 140 μm and 10 with 70 μm pixels were successfully implanted subretinally in 27 rats (see Methods ): 12 wild-type (Long-Evans) and 15 animals with retinal degeneration (RCS), as listed in Table 1 . Follow-up with optical coherence tomography (OCT) imaging revealed gradual resolution of mild retinal oedema or retinal detachment within the first few weeks after implantation. 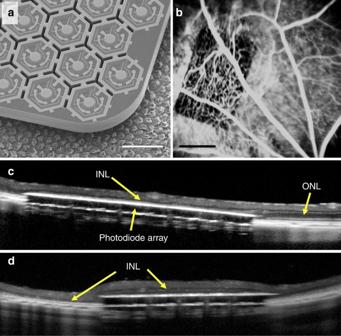Figure 2: Photodiode arrays in the eye. (a) Scanning electron micrograph of a photodiode array with 70 μm pixels above the RPE in a porcine eye. Scale bar, 70 μm. (b) Fluorescein angiography 10 days after subretinal implantation of the photodiode array in WT rats shows good perfusion over the implant with no staining or leakage. Scale bar, 500 μm. (c) OCT of a WT rat 12 weeks after subretinal implantation. INL (pointed by the arrow) is in close proximity to the implant, with no evidence of retinal oedema or injury. Photoreceptor layer above the implant is missing due to prolonged separation from the RPE. Implant appears 77 μm thick instead of actual 30 μm due to much higher refractive index of silicon (n≈3.6) than that of ocular tissues (n≈1.4). (d) OCT of an RCS rat 7 days after implantation. INL (indicated by the arrow) is in close proximity to the implant. As expected, due to retinal degeneration, there is no photoreceptor layer. Figure 2c depicts a typical OCT image of an implant in the subretinal space. Because of the much higher refractive index of silicon ( n ≈3.6) than that of ocular tissues ( n ≈1.4), the implant appears almost three times thicker than it actually is: 77 μm instead of 30 μm. The upper surface of the implant is in close proximity to the INL, where the target neurons for electrical stimulation (bipolar cells) reside. Fluorescein angiography revealed normal vasculature and good perfusion of the retina overlying the implants ( Fig. 2b ). As the Si array blocks visible light, there is no fluorescent background from the choroid, which improves visibility of the retinal vasculature above the implant. As expected, the presence of the implant between the retinal pigmented epithelium (RPE) and photoreceptors in wild-type (WT) animals caused gradual degradation and disappearance of the photoreceptors above the implant while leaving the adjacent retina unaffected ( Fig. 2c ). In 7 out of 12 cases of WT rats, we found fluorescent deposits above the implant, beginning a few weeks following the implantation. These are likely associated with degeneration of photoreceptors detached from the RPE by the implant. In RCS rats, diffuse autofluorescence was distributed over the whole retina, as part of the degenerative process [24] . There were no cases of infection or inflammatory reaction during the 6 months of follow-up. Table 1 The range of stimulation thresholds for different pixel sizes. Full size table Figure 2: Photodiode arrays in the eye. ( a ) Scanning electron micrograph of a photodiode array with 70 μm pixels above the RPE in a porcine eye. Scale bar, 70 μm. ( b ) Fluorescein angiography 10 days after subretinal implantation of the photodiode array in WT rats shows good perfusion over the implant with no staining or leakage. Scale bar, 500 μm. ( c ) OCT of a WT rat 12 weeks after subretinal implantation. INL (pointed by the arrow) is in close proximity to the implant, with no evidence of retinal oedema or injury. Photoreceptor layer above the implant is missing due to prolonged separation from the RPE. Implant appears 77 μm thick instead of actual 30 μm due to much higher refractive index of silicon ( n ≈3.6) than that of ocular tissues ( n ≈1.4). ( d ) OCT of an RCS rat 7 days after implantation. INL (indicated by the arrow) is in close proximity to the implant. As expected, due to retinal degeneration, there is no photoreceptor layer. Full size image To assess potential effect of the implant on neural retina, the thickness of the inner retinal layers (from the INL up to the inner limiting membrane (ILM)) was measured in 9 WT rats over the follow-up period using OCT. No significant change in thickness of the inner retina has been observed: average thickness above the implant changed from 58 μm during the first month after implantation to 54 μm at the end of the follow-up period (matched t -test, P =0.4). Average inner retinal thickness away from the implant decreased from 64 to 58 μm, but the difference also was not statistically significant (matched t -test P =0.2). In a few animals, we observed gradual retinal thinning or decrease in vascularization along one of the longer edges of the implant. This effect is probably induced by elevation of the middle part of the rectangular implant above the RPE in a spherically shaped eyeball. This may not be a problem in human eyes, as the curvature of the eyeball is about five times larger, and this issue can be avoided using arrays of a round shape rather than rectangular. Visual-evoked potentials Following successful subretinal implantation, trans-cranial screw electrodes were placed over the primary visual cortex (see Methods ) and animals were observed for another week before recording VEP signals. Three experiments were performed as controls. First, to check for natural sensitivity of the rat retina to infrared light, near-IR (NIR) pulses were applied to the same spot size on the retina away from the implant at maximum irradiance and pulse duration: 20 mW mm −2 and 10 ms. No VEP responses were observed. Second, to check for possible direct effect of the stimulation current on the brain, retrobulbar injection of Lidocain 2% was applied to block signal transduction via optic nerve. This resulted in complete disappearance of VEP signals for both, the visible light and NIR. Third, NIR stimulation was applied to two deceased rats (which showed robust eVEP when alive), and it elicited no VEP, just a short stimulation artifact, similar to the one depicted in Fig. 3c (*). 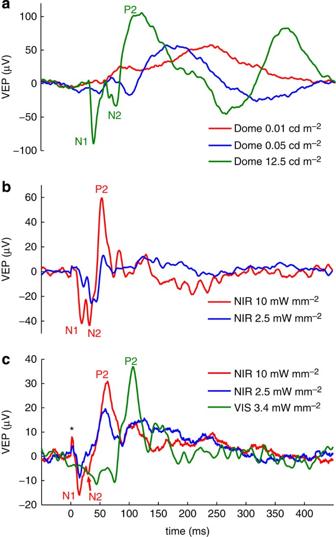Figure 3: Cortical responses in WT (normally sighted) animals. (a) VEP of the WT animal in response to white light at various luminance levels provided by dome stimulator. With brighter stimuli, the VEP amplitude increases and latency decreases. (b) NIR stimuli over the implant with 70 μm pixels elicited a prompt eVEP with similar structure but significantly shorter latencies: N1 and P2 at 19 ms and 53 ms, respectively. Amplitude of both N1 and P2 increased at higher irradiances. This recording was performed 4 months after implantation. (c) VEP (green) elicited by visible (635 nm) light projected onto 1 mm spot away from the implant and eVEP (blue and red) were recorded in the same WT animal implanted with 280 μm pixels array. eVEP were recorded in response to 4 ms NIR stimuli at peak irradiances of 2.5 (blue) and 10 mW mm−2(red), repeated at 2 Hz. A short artifact caused by the photovoltaic current is indicated by *. Figure 3: Cortical responses in WT (normally sighted) animals. ( a ) VEP of the WT animal in response to white light at various luminance levels provided by dome stimulator. With brighter stimuli, the VEP amplitude increases and latency decreases. ( b ) NIR stimuli over the implant with 70 μm pixels elicited a prompt eVEP with similar structure but significantly shorter latencies: N1 and P2 at 19 ms and 53 ms, respectively. Amplitude of both N1 and P2 increased at higher irradiances. This recording was performed 4 months after implantation. ( c ) VEP (green) elicited by visible (635 nm) light projected onto 1 mm spot away from the implant and eVEP (blue and red) were recorded in the same WT animal implanted with 280 μm pixels array. eVEP were recorded in response to 4 ms NIR stimuli at peak irradiances of 2.5 (blue) and 10 mW mm −2 (red), repeated at 2 Hz. A short artifact caused by the photovoltaic current is indicated by *. Full size image Typical eVEP response to photovoltaic stimulation was characterized by two early negative components at 15–21 ms (N1) and 35–41 ms (N2), followed by two positive peaks at 30–35 ms (P1) and 55–60 ms (P2). A later smaller positive peak (P3) typically had latency>100 ms ( Fig. 3b ). VEP response to the natural photopic stimuli was first obtained with the full-field uniform white illumination using the dome ( Fig. 3a ), and then with a 1 mm spot (same size as the implant) of red (635 nm) light projected from the slit lamp away from the implant. With both, the full-field and the spot illumination, the VEP had generally similar structure (N1, P1, N2, P2, P3), but was delayed compared with the response to photovoltaic stimulation ( Fig. 3c ). Though the latency of N1 decreased with increased irradiance (Fig. 5d), the shortest latency observed was 40 ms—about 20 ms later than the first negative peak in photovoltaic stimulation. This difference is likely due to the fact that electrical stimulation elicits responses from the inner retinal neurons, bypassing the phototransduction process in the retina, which can take up to several tens of milliseconds [25] . It should be noted that much brighter light at 635 nm was required to elicit VEP responses equivalent in amplitude to those from the full-field white-light illumination (dome). This difference is likely to be due to at least two factors: much lower sensitivity of rodent retina at 635 nm as compared with white light [26] , and smaller area of the illuminated retina. It is quite possible that red light scattered from the small illuminated spot activated the whole retina in the eye. The eVEP recorded from RCS rats had similar structure to that of the WT rats, as illustrated in Fig. 4b for RCS rat implanted with a 70-μm pixels array. However, the VEP in response to white light in RCS rats was very weak and slow, with no significant N1, even with very bright full-field stimuli ( Fig. 4a ). Visible light stimulation with 1 mm spot did not elicit any detectable VEP. 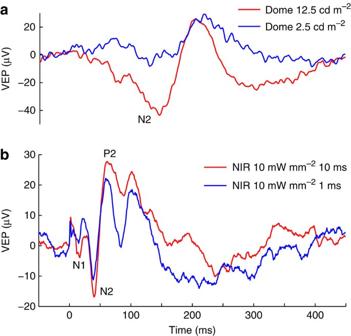Figure 4: Cortical responses in animals with degenerate retina. VEP (a) and eVEP (b) recording from an RCS rat (age 17 weeks) implanted with 70 μm pixel-size array. (a) VEP traces in response to full-field (dome) white light stimuli at two irradiance levels show slow and weak response even at high illumination. N1 latency is 70 ms and P wave more than 200 ms (compared with faster and stronger response in WT rat, shown inFig. 3a). (b) eVEP in the same rat in response to NIR stimulation over the implant at 10 mW mm−2, with 1 and 10 ms pulses. Longer pulse duration elicited stronger eVEP response. Figure 4: Cortical responses in animals with degenerate retina. VEP ( a ) and eVEP ( b ) recording from an RCS rat (age 17 weeks) implanted with 70 μm pixel-size array. ( a ) VEP traces in response to full-field (dome) white light stimuli at two irradiance levels show slow and weak response even at high illumination. N1 latency is 70 ms and P wave more than 200 ms (compared with faster and stronger response in WT rat, shown in Fig. 3a ). ( b ) eVEP in the same rat in response to NIR stimulation over the implant at 10 mW mm −2 , with 1 and 10 ms pulses. Longer pulse duration elicited stronger eVEP response. Full size image To evaluate whether stimulation of the RGCs by subretinal photovoltaic array is mediated by the inner retinal neurons, a cocktail of synaptic transmission blockers was injected intravitreally in four WT rats. Such injections resulted in immediate disappearance of the cortical responses to both, the visible and NIR light (10 ms, up to 10 mW mm −2 , Supplementary Fig. S2a ), and both responses returned to normal the next day. This result suggests involvement of the inner retinal neurons and retinal network in subretinal stimulation. To control for potential effects of the intraocular pressure rise, intravitreal injections of a similar volume of fluid without the active ingredients have been performed, and they did not affect cortical responses ( Supplementary Fig. S2b ). The normalized VEP amplitude increased with peak irradiance over four orders of magnitude of the visible light brightness, following a characteristic sigmoid curve ( Fig. 5c ). Over the central two orders of magnitude (0.05–2.5 cd m −2 ), the signal increased logarithmically. The eVEP response also increased logarithmically with peak irradiance over two orders of magnitude of the NIR irradiance ( Fig. 5a ), with no significant difference between the animal types. However, while N1 latency in VEP elicited by visible light significantly decreased with increased illumination ( Fig. 5d ); in eVEP elicited by NIR, the N1 latency did not vary with irradiance ( Fig. 5b ). Normalized eVEP could also be modulated by pulse duration while keeping the irradiance constant ( Fig. 6a ) and showed a logarithmic increase with pulse duration from 1 to 10 ms. In RCS group, the rise with pulse duration ( Fig. 6a , red line) was slower than in the WT animals ( Fig. 6a , blue line). Similarly, VEP elicited by visible light in WT animals increased in amplitude logarithmically with pulse duration ( Fig. 6b ). 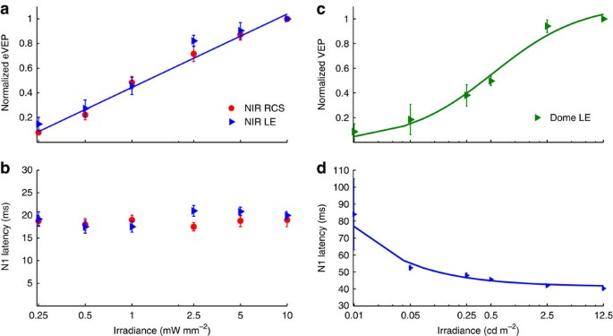Figure 5: VEP amplitude and latency as a function of peak irradiance for NIR and visible stimuli. (a) The eVEP amplitude (N1–P2), normalized to response at 10 mW mm−2, and averaged for 7 WT and 7 RCS rats is plotted as a function of peak irradiance. Pulse duration was held constant at 10 ms. The eVEP amplitude increased logarithmically with peak irradiance, with no significant difference between the two animal types. (b) N1 latency in the same eVEP recordings did not vary with irradiance, and was very similar in the two animal groups. (c) Normalized VEP amplitude in WT rats, in response to white light full-field stimuli, averaged over six animals, and plotted as a function of the peak irradiance. For averaging between the animals, the VEP amplitude was normalized to the response at maximum irradiance. Error bars represent the s.e.m. (d) N1 latency as a function of the peak irradiance in the same data set. Figure 5: VEP amplitude and latency as a function of peak irradiance for NIR and visible stimuli. ( a ) The eVEP amplitude (N1–P2), normalized to response at 10 mW mm −2 , and averaged for 7 WT and 7 RCS rats is plotted as a function of peak irradiance. Pulse duration was held constant at 10 ms. The eVEP amplitude increased logarithmically with peak irradiance, with no significant difference between the two animal types. ( b ) N1 latency in the same eVEP recordings did not vary with irradiance, and was very similar in the two animal groups. ( c ) Normalized VEP amplitude in WT rats, in response to white light full-field stimuli, averaged over six animals, and plotted as a function of the peak irradiance. For averaging between the animals, the VEP amplitude was normalized to the response at maximum irradiance. Error bars represent the s.e.m. ( d ) N1 latency as a function of the peak irradiance in the same data set. 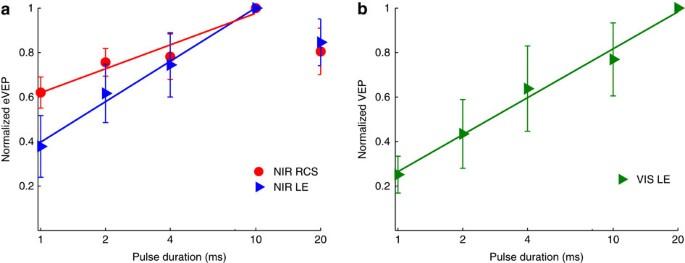Figure 6: VEP amplitude as a function of pulse duration. (a) eVEP amplitude (N1–P2), normalized to response at 10 ms, and averaged for 6 WT and 4 RCS rats. eVEP amplitude increased logarithmically with pulse duration from 1 to 10 ms, and slightly decreased at 20 ms. In the RCS group, the rise with pulse duration (red line) was smaller than in the WT animals (blue line). (b) Average VEP amplitude elicited by a 1 mm spot of visible light (635 nm), in 6 WT animals, as a function of pulse duration, normalized to its maximum value. Error bars represent the s.e.m., dashed lines represent logarithmic fit. Full size image Figure 6: VEP amplitude as a function of pulse duration. ( a ) eVEP amplitude (N1–P2), normalized to response at 10 ms, and averaged for 6 WT and 4 RCS rats. eVEP amplitude increased logarithmically with pulse duration from 1 to 10 ms, and slightly decreased at 20 ms. In the RCS group, the rise with pulse duration (red line) was smaller than in the WT animals (blue line). ( b ) Average VEP amplitude elicited by a 1 mm spot of visible light (635 nm), in 6 WT animals, as a function of pulse duration, normalized to its maximum value. Error bars represent the s.e.m., dashed lines represent logarithmic fit. Full size image Stimulation thresholds were determined as the minimum stimuli peak irradiance eliciting a VEP signal with amplitude 3 s.d. above the noise level (see detailed description in Methods). Table 1 lists the average values and the range of stimulation thresholds for various pixel sizes with 4- and 10-ms pulse durations. The lowest threshold in this series was 0.25 mW mm −2 at 4 ms, observed in a WT animal implanted with 140 μm pixel array. On an average, the thresholds increased with decreasing pixel size: from 0.43 mW mm −2 with the 280 μm pixels to 1 mW mm −2 with the 140 μm arrays, and to 2.1 mW mm −2 with the implants having 70 μm pixels. Thresholds decreased, on average, by a factor of 1.8 when pulse duration increased from 4 to 10 ms. There was no statistically significant difference between the stimulation thresholds in RCS and in WT rats. As can be seen from comparison of the Figs 3 and 4 , the shape and amplitude of the eVEP in RCS rats was quite similar to those of the WT responses. Simultaneous pulsed stimulation of the retina with patterns representing visual scenes is more similar to stroboscopic vision rather than to the natural continuous illumination. At sufficiently high frequencies, the pulsed stroboscopic representation fuses into a continuous perception [27] . We assessed potential differences in frequency response to pulsed electrical and visible light stimuli by measuring the amplitude of VEP (N1 to P2) at various pulse-repetition rates ( Fig. 7a ). VEP amplitude, in response to electrical stimulation, decreased with increasing frequency from 2 to 20 Hz—similar to the visible light-induced response ( Fig. 7b ). From 20 to 40 Hz, the visible response continued to decrease, whereas the eVEP did not change as much. The difference becomes more profound taking into account the decrease of the photovoltaic current with frequency, as measured by the amplitude of the stimulation artifact ( Fig. 7b ). As expected from the RC circuit with a resistance-limited discharge rate, photovoltaic current decreased exponentially with frequency [21] . 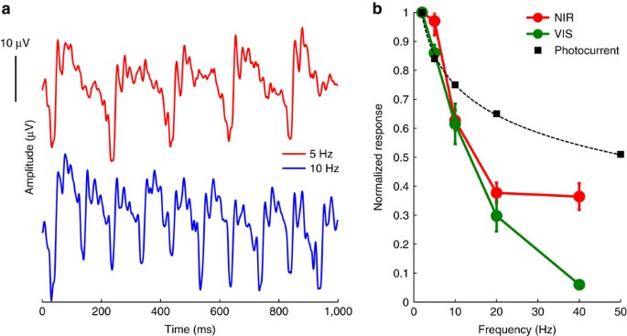Figure 7: VEP elicited by 1 mm visible light spot on the retina. (a) Robust VEP response to 5 (upper trace) and 10 Hz (lower trace) NIR stimulation in a WT rat. (b) Amplitude of VEP in response to NIR (red, averaged forn=18) and visible (green, averaged forn=6) stimuli at frequencies of 2–40 Hz. Error bars represent s.e.m. Blue dashed line depicts the frequency response of the photocurrent from the implant. Figure 7: VEP elicited by 1 mm visible light spot on the retina. ( a ) Robust VEP response to 5 (upper trace) and 10 Hz (lower trace) NIR stimulation in a WT rat. ( b ) Amplitude of VEP in response to NIR (red, averaged for n =18) and visible (green, averaged for n =6) stimuli at frequencies of 2–40 Hz. Error bars represent s.e.m. Blue dashed line depicts the frequency response of the photocurrent from the implant. Full size image Electrophysiological responses of the WT and RCS rats remained very robust during the whole 6-month-long follow-up period. For example, the VEP responses shown in Fig. 3b were recorded 4 months after implantation. However, on average, the stimulation thresholds with 10 ms pulses increased by 58% over the follow-up period. As these implants were not protected by SiC coating for long-term stability, erosion of the silicon nitride antireflection coating of the chips [23] in the body was expected to start affecting their performance over several months of implantation. Increase in the stimulation thresholds could also be attributed to retinal changes or to corneal oedema developed over time in some animals due to irritation by the gel and contact lens. Robust eVEP responses to photovoltaic subretinal stimulation suggest that visual information elicited by the implant in the retina arrives at the visual cortex. Cortical responses could be modulated by both light intensity and pulse width, similar to modulation of the RGC responses in vitro [19] . Like with visible light stimulation, the RGC-spiking rate was gradually increasing with stronger electrical stimuli, indicating preservation of the retinal network signal processing, at least to some extent [19] . Gradual increase in eVEP with stronger stimuli for both, visible light and subretinal electric pulses, shown in the current study, further illustrate similarity of the visual system responses to pulsed visible light and subretinal electrical stimulation. Both, pulse duration and brightness control can be used for modulation of the image in NIR projection systems. Liquid crystal displays allow modulation of light intensity with constant pulse duration in each pixel, while digital light processing micro-mirror arrays (also known as digital micro-mirror device) allow pulse duration control with constant light intensity in each pixel. The latter approach should enable rapid sequential activation of pixels, potentially reducing cross-talk between adjacent electrodes [18] . In addition, the image can be controlled with spatial light modulators, providing higher throughput and allowing amplitude or duration modulation in each pixel [28] . Stimulation thresholds increased with decreasing pixel size, which may be due to several reasons: shallower penetration of electric field with smaller electrodes (as return electrode is closer), lower fraction of open silicon for light collection, or reduced number of neurons affected by stimulation with smaller electrodes. With smallest pixels (70 μm), the average stimulation threshold with 4 ms pulses were 3.8 mW mm −2 , 53 times below the ocular safety limit for single-pulse exposure (200 mW mm −2 at 905 nm) [21] , [19] . With repetition rate of 7.5 Hz, the perceptual limit of subretinal stimulation in human patients [16] , the average retinal irradiance is about 0.11 mW mm −2 , 47 times lower than the ocular safety limit for prolonged exposures (5.2 mW mm −2 ) [21] . Current implants generate cathodic-first electric pulses. Anodic pulses have lower stimulation thresholds in subretinal placement: by a factor of 2–7 (ref. 29 ). Lower stimulation thresholds are therefore expected with anodic version of the photovoltaic array. Latency (N1) of the visible light-evoked responses decreases with increasing irradiance due to reduced integration time in photoreceptors [25] , [30] . In our set-up, it reached 35 ms at highest measured brightness level ( Fig. 3 ). Phototransduction is bypassed during electrical stimulation of the inner retinal neurons, resulting in an earlier appearance of the N1 peak, by at least 15 ms, compared with visible light stimulation. Direct stimulation of RGCs in the epiretinal approach, bypassing the inner retinal neurons, also resulted in shorter VEP latencies, compared with visible light responses [31] . Similarity in decrease of the VEP amplitude with increasing frequency for visible and photovoltaic stimulation below 20 Hz indicates that it is governed by processes other than phototransduction. A very similar VEP decrease with higher frequencies was also reported for epiretinal [31] and optic nerve stimulation [32] up to 10 Hz. However, at frequencies higher than 20 Hz, the eVEP did not decrease as rapidly as visual light response. This difference is likely due to phototransduction delay, as its time constant is on the order of 30–40 ms. Disappearance of the cortical responses upon intravitreal application of synaptic blockers suggests that retinal stimulation by photovoltaic subretinal array originates in the inner retinal neurons, and is mediated by the retinal neural network. This conclusion is also supported by the similarity between the frequency dependence of the network-mediated stimulation of RGCs in vitro [33] , [34] and the eVEP decrease with frequency in the present study. However, it should be noted that depending on pulse amplitude, polarity and electrode geometry, subretinal stimulation can result in both, the network-mediated and direct responses of RGCs, with latency difference as low as 2–3 ms (ref. 35 ). Similarity of the implant-induced VEP waveforms to the visible light response, including the late components such as P2 and P3, suggests that retinal response to both types of stimuli arrived to the thalamus and visual cortex. Nevertheless, processing of the electrically induced information in the primary visual cortex and in the higher visual areas might be affected by the highly synchronized response to pulsed electrical stimuli, lack of latency dependence on stimulus intensity, lack of selectivity in the ‘on’ and ‘off’ pathways and absence of many other aspects of natural retinal signal processing. Localization of the stimuli in front of the electrode array is determined by the size of the active electrodes and geometry of the return electrodes. In the current implant design, circumferential return electrodes in each pixel are connected to each other. Larger area of the connected return electrodes in this arrangement helps reducing the impedance and thereby the stimulation threshold. However, this also causes spread of electric current over areas larger than one pixel and may degrade resolution. This tradeoff between stimulation thresholds and resolution of the arrays should be carefully studied and optimized. Investigation of the resolution of retinal stimulation in vitro is complicated by wide variety of sizes of the RGC-receptive fields. Studies of the resolution in vivo could be performed with either behavioural tests (for example, optokinetic response) or with VEP response to moving patterns. Small implant size and somewhat random positioning of the chip in a small eye make behavioural tests of visual acuity in rats quite challenging. VEP response to alternating patterns is a very promising approach, as long as it is carefully controlled for potential artifacts, including constant average irradiance for all patterns on the implant, and pulse-repetition rate exceeding the flicker fusion frequency. Alternating patterns projected with stroboscopic illumination induce a mixed VEP response to both, each pulse and to the pattern movement. Because of the slower decrease of VEP at higher frequencies with photovoltaic stimulation ( Fig. 7b ), the reliable discrimination between the VEP response to slow moving patterns and responses to each flash may require higher repetition rates of stimulation than those used with visible light. The issue is further complicated by the decreasing implant efficiency with increasing frequency ( Fig. 7b ). Future studies will also explore the optimal spatiotemporal protocols of retinal stimulation by allowing sequential activation of pixels and thereby reducing the stroboscopic perception of single pulses. Separation of the retina from RPE above the implant resulted in local degeneration of the photoreceptors in WT animals, while sparing the inner retinal layers and adjacent retina, which remained stable over the follow-up period ( Fig. 2c ). Retinal degeneration above the implant may explain the fact that stimulation thresholds in WT and RCS animals were similar in vivo , while in vitro the RCS rat retina had stimulation thresholds twice higher than that of the WT animals [19] . This effect may serve a convenient model of local retinal degeneration, obviating the need for genetic models potentially affecting many other functions of the animal. Erroneous retinal rewiring during degeneration [36] is one of the major concerns with the network-mediated stimulation in subretinal approach to retinal prosthetics. It should be noted however, that subretinal stimulation in patients blinded by retinitis pigmentosa (light perception only) resulted in visual acuity up to 20/550 (ref. 16 ). On the other hand, it was also noted that stimulation thresholds in human patients increased with progression of retinal degeneration, which indicates a possibility of better results with implantation at earlier stages of the disease [37] . One intriguing possibility of chronic stimulation is restorative retinal rewiring in response to functional stimulation. In conclusion, we demonstrated that the small implant size and lack of wires make photovoltaic arrays easy to implant, even in the eyes as small as in rats. The implants were well tolerated in the subretinal space, and stable over the 6 months follow-up. Robust cortical responses could be broadly modulated by irradiance, pulse duration and frequency, with stimulation thresholds well below the ocular safety limits. eVEP had generally similar shape and amplitude to the visually evoked responses, although the latency of the first peak was shorter in eVEP due to lack of phototransduction. eVEP amplitude scaled with NIR irradiance, frequency and pulse duration similarly to the response to pulsed visible light. Similarities in characteristics of the cortical response to electrical subretinal stimulation and pulsed visible light provide encouraging reassurance in feasibility of the photovoltaic approach to retinal prosthetics. The modularity and scalability of the photovoltaic arrays to a large number of pixels offers a promising approach to functional restoration of sight in patients suffering from blinding degenerative retinal diseases. Implant fabrication The fabrication process of the implant is described in detail elsewhere [23] . Briefly, the array was fabricated on lightly boron-doped silicon-on-insulator wafers. The 30-μm thick device can absorb a significant fraction (~70%) of the NIR light, while still being thin enough to be implanted underneath the retina. Each pixel has three photodiodes connected in series between the central active and circumferential return electrodes. Pixels are separated by 5-μm-wide trenches to improve electrical isolation and to allow nutrient flow through the implant. Photodiodes convert light into electric current with efficiency of about 0.36 A/W/diode [23] . Electrodes are coated with iridium oxide to maximize the charge injection capacity. Animal care and surgical procedures All animal care and experiments were carried out in accordance with the ARVO guidelines for the Use of Animals in Ophthalmic and Vision Research and approved by the Stanford Administrative Panel on Laboratory Animal Care. Long-Evans adult WT rats were purchased from Charles River (Wilmington, MA, USA). Rats with retinal degeneration were obtained from the Royal College of Surgeons (RCS) colony maintained at Stanford Animal facility [38] . All animals are housed in a 12-h light/12-h dark cycle with food and water ad libitum . Animals were operated on at a mean age of 79 days (range 50–120 days), and recording starting 2 weeks after the implantation. Subretinal implantation technique was similar to the previously reported one by our group [39] . Briefly, a 1.5-mm incision was made through the sclera and choroid 1.5 mm posterior to the limbus, and the implant was placed into the subretinal space using a custom-made implantation tool. The sclera and conjunctiva were sutured with nylon 10-0 and topical AB (polymixin B) was applied on the eye post operatively. The number of animal used in each group is shown in Table 1 . Overall results of 27 animals are reported in this paper. In vivo imaging The anatomical integration of the device into the subretinal space was evaluated by OCT (HRA2-Spectralis, Heidelberg Engineering, Heidelberg, Germany) in consecutive examinations beginning 1 week after surgery. HRA2-Spectralis system (cSLO at 488-nm blue excitation and 500 nm green emission filter) was used for both autofluorescence imaging and for fluorescein angiography, following intraperitoneal injection of 0.2 mg/kg fluorescein sodium diluted in balanced salt solution. The thickness of inner retina (from INL to ILM) was evaluated over a follow-up period of 10–23 weeks (average 20 weeks). The outer retinal layers (photoreceptors and OPL) degenerated over time as part of the disease in RCS rats, and due to mechanical separation from the RPE in the WT rats. Implantation of the VEP electrodes Three skull screw electrodes were implanted similar to the previously published technique [40] and secured in place with cyanoacrylate glue and dental acrylic. Two electrodes were placed over the visual cortex of both hemispheres, 4 mm lateral from midline, 6 mm caudal to the bregma. One reference electrode was implanted 2 mm right to the midline and 2 mm anterior to the bregma. Nose and tail needle electrodes served as a reference and the ground, respectively. Anaesthesia during recording Rats were anaesthetized with a mixture of ketamine (0.375 mg kg −1 ) and xylazine (0.125 mg kg −1 ) injected intraperitoneally. The following steps were taken to assure steady anaesthesia: spontaneous eye movements and respiratory pattern were checked periodically; additional injections of the 50% of the initial dose were administered every 40 min, or as needed, and recording sessions were limited to 90 min per session. A heating pad was used to maintain the body temperature at 37.5±0.5 °C. Electrophysiological recording were conducted with a dim-room illumination of 250 nW cm −2 . Stimulation The laser projection system included NIR (915 nm) and visible light (635 nm) laser diodes coupled into a 1-mm optical fibre mounted on a slit lamp (Zeiss SL–120). Following the pupil dilation and eye retraction for optimal alignment of the implant, a small glass cover slip with viscoelastic material was applied to optically flatten the rat cornea and enable imaging of the subretinal implant and focusing of the laser beam. Position of the beam during the experiments was monitored by CCD camera mounted on the same slit lamp. The 635-nm laser was used for aiming and as a visible light source for VEP recordings. NIR stimulation was applied with pulse durations ranging from 1 to 20 ms, and peak irradiances from 0.05 to 10 mW mm −2 . Full-field white stimuli were provided by the Ganzfeld dome (Espion E2, Diagnosys, Westford, MA, USA) using flashes at 2 Hz. In all, 250–500 trials were averaged for each set of parameters. Irradiance was varied in the range of 0.01–12.5 cd m −2 . VEP recording and analysis VEP signals were recorded by Espion E2 system (Diagnosys). Data was acquired at 1 kHz with no temporal filtering. At least 500 trials were averaged for each result. A threshold VEP response was defined as 3 s.d. above the noise level during the first 100 ms after the stimulus, as illustrated in Supplementary Fig. S1 .The noise level was defined as the RMS value calculated from the data recorded during the 50 ms preceding the stimuli. The frequency response of the VEP was studied with NIR pulses of 10 ms duration and 10 mW mm −2 peak irradiance and visible pulses of 10 ms duration and 3.4 mW mm −2 irradiance, applied at 2, 5, 10, 20 and 40 Hz. Amplitude of the response was measured from the minimum value at N1 peak to the maximum at P2 peak (N1–P2) for each stimuli frequency and normalized, for each animal, by the amplitude at 2 Hz. Blocking retinal synaptic transmission Cortical responses in response to visible and NIR light were recorded before, 30 min after and the day following intravitreal injection of synaptic blockers cocktail. Final in-vitreous concentration of the blockers were calculated as 0.8 mM L-AP7, 0.2 mM NBQX, 0.4 mM strychnine, 0.8 mM L-AP4 and 0.32 mM picrotoxin, assuming vitreous volume of 50 μl (ref. 41 ). To control for potential effects of the intraocular pressure rise due to injection, intravitreal injections of a similar volume of fluid without the active ingredients have also been performed. Recording photocurrent response in vitro The photodiode array was placed in buffered saline solution (BSS) and illuminated by pulses of NIR light (5 ms, 10 mW mm −2 , 905 nm) projected through the BSS layer. Electrical signals in the medium were measured using a glass pipette microelectrode placed above the implant. The recorded signal was amplified with a bandpass filter of 1 Hz–100 kHz (Multiclamp 700A, Molecular Devices, USA) and digitized (Digidata 1440, Molecular Devices). The peak amplitude of the recorded current spike, normalized by its value at 2 Hz, was used to quantify the relative electrical response at various pulse-repetition rates. How to cite this article: Mandel, Y. et al . Cortical responses elicited by photovoltaic subretinal prostheses exhibit similarities to visually evoked potentials. Nat. Commun. 4:1980 doi:10.1038/ncomms2980 (2013).